Arl3 and LC8 regulate dissociation of dynactin from dynein Cytoplasmic dynein acts as a motor for the intracellular retrograde motility of vesicles and organelles along microtubules. However, the regulatory mechanism underlying release of dynactin bound cargoes from dynein motor remains largely unknown. Here we report that ADP-ribosylation factor-like 3 (Arl3) and dynein light chain LC8 induce dissociation of dynactin from dynein. Immunoprecipitation and microtubule pull-down assays revealed that Arl3(Q71L) and LC8 facilitated detachment of dynactin from dynein. We also demonstrated Arl3(Q71L) or LC8-mediated dynactin release from a dynein–dynactin complex through trace experiments using quantum dot (Qdot)-conjugated proteins. Furthermore, we disclosed interactions of Arl3 and LC8 with dynactin and dynein, respectively, by live-cell imaging. Finally, knockdown (KD) of Arl3 and LC8 by siRNA induced abnormal localizations of dynein, dynactin and related organelles. Our findings uncovered the surprising functional relevance of GTP-bound Arl3 and LC8 for the unloading regulation of dynactin-bound cargo from dynein motor. Cytoplasmic dynein is a multisubunit molecular motor that uses ATP hydrolysis to participate in microtubule-based retrograde transport [1] , [2] . Within cells, cytoplasmic dynein transports numerous cargoes, including organelles, proteins and RNAs, and is required for cell division [1] , [2] . Cytoplasmic dynein consists of heavy chain (HC), intermediate chain (IC), light IC and light chain (LC) subunits, all of which exist as homodimers in the fully formed complex. In addition, cytoplasmic dynein interacts with several proteins that do not belong to the dynein complex itself, but are crucial for adapting the motor to its cellular function including dynactin, LIS1 and NDEL1 (refs 3 , 4 , 5 ). These factors contribute to many dynein functions, and in the cases of NDEL1 and LIS1 their inhibition or depletion is phenotypically similar to a complete loss of dynein function [6] , [7] . Dynactin was identified as an activator of dynein-mediated, minus end-directed vesicle transport in vitro [3] , [4] . The dynactin complex comprises 11 different subunits, including the largest subunit, p150 Glued , p50 and a filament of actin-related protein 1 (Arp1). Importantly, dynactin has been found to be essential for nearly every cellular function of cytoplasmic dynein, such as cargo loading, dynein localization and maintaining processivity [5] , [8] . For example, Arp1 filament of dynactin binds to βIII spectrin, a filamentous protein that is found on the cytosolic surface of the Golgi and other cellular membranes [9] . Dynactin p150 Glued is also an important component for connection of a dynactin complex with a dynein motor. The second coiled-coil domain of p150 Glued aa 925–1050 on coiled coil 2 (CC2) contains a conserved actin-binding motif that has been proposed to bind the Arp1 filament directly [10] . Moreover, p150 Glued aa 217–548 on CC1 interacts with amino-terminal fragments of the dynein IC (DIC) [11] and the aa 600–811 was also reported to bind full-length DIC [12] , but the latter binding is controversial [13] . Thus, p150 Glued functions as a hub for connection of dynein with cargo. Interaction of dynein and dynactin is exquisitely regulated for directional and accurate transports of cellular components, which highlights the importance of understanding how dynein–dynactin interaction is spatially and temporally controlled. Recently, G protein-mediated regulation of motor–cargo assembly are emerging. Rab GTPases constitute the largest family of small GTPases, which are reversibly associated with membranes by hydrophobic geranylgeranyl groups that are attached to one or two carboxy-terminal Cys residues, and this is intrinsic to their role in regulating membrane traffic [14] . Through their indirect interactions with coat components, motors and SNAREs, the Rab GTPases serve as multifaceted organizers of almost all membrane-trafficking processes in eukaryotic cells. For example, Rab3 plays a critical role in the loading and unloading of synaptic vesicle precursors [15] . Rab11A regulates endosomal trafficking events by associating with kinesin-2 (ref. 16 ). Rab27A and Rab27B associate with kinesin-1 to regulate axonal transport of neurotrophin receptor-containing vesicles [17] . Members of the ADP-ribosylation factor (Arf) also regulate membrane traffic and organelle structure by recruiting cargo-sorting coat proteins, modulating membrane lipid composition and interacting with regulators of other G proteins [18] , [19] . The Arf family contains secretion-associated and Ras-related 1 (Sar1), Arf1-6 and a number of Arf-like (Arl) proteins that are similar to Arfs but more distantly related. In this family, the functions of Sar1 and Arf1 are well established, but the roles of most of the Arl proteins are less well characterized. We previously reported that Rab6a(Q72L) dissociates LIS1 from a LIS1–dynein complex, followed by activating dynein movement in in vitro microtubule gliding assays [20] . One remaining challenge is to address the machinery that regulates unloading of cargoes from dynein. Although the loading/unloading mechanisms for kinesin motor have been intensively investigated, how dynein regulates loading/unloading cargoes is beginning to be determined. In this study, we demonstrate that dissociation of dynactin from dynein is regulated by ADP-ribosylation factor-like 3 (Arl3) and LC8. Arl3 and LC8 bind dynactin p150 Glued and dynein HC, respectively. In particular, LC8 and Arl3 exhibit similar subcellular localizations in mouse embryonic fibroblast (MEF) cells that are characterized by gradient distribution carrying a peak at the perinuclear region. Presumably, regulation of disassembly of dynein–dynactin complex by LC8 and Arl3 will ensure the unloading of cargo from a dynein motor. Our findings provide new insights into the underlying mechanisms by which the unloading of cargo from dynein is regulated. Arl3 and LC8 induce dissociation of dynactin from dynein At the beginning of this study, we explored the regulatory factors that could release dynactin from a dynein motor. Recently, we demonstrated that Rab6a is an essential factor to activate dynein and to load cargo at the plus-end of microtubules [20] . We assumed that other small G proteins may be involved in the unloading process. The Rab and Arf GTPases are members of two of the Ras-related subfamilies that function in regulating vesicle trafficking, starting from regulating the formation of vesicles on donor membranes and directing trafficking specificity to and facilitating vesicle docking on target membranes [14] , [21] . In particular, members of Arf family, including the Arl proteins and Sar1, regulate membrane traffic and organelle structure in the centrosomal region of the cell [18] . Therefore, we screened Arf/Arl family proteins to identify a candidate that is involved in disassembly of dynein–dynactin complexes by microtubule pull-down assays. As shown in Supplementary Fig. 1a,b , GTP-bound Arl3(Q71L) seems to be apparently effective in disassembly of the dynein from microtubule-bound dynactin. Ctp was isolated as a P[lacW] insertion in fruit fly [22] , which encodes LC8 family members of dynein LCs (DYNLL1 and DYNLL2 in vertebrates). Investigation of genetic interaction of ctp suggests that LC8 functionally interacts with dynein HC and dynactin p150 Glued (FlyBase: http://flybase.org ). In addition, nudG encodes a homologue of LC8 (ref. 23 ), which is one of the nud genes involved in nuclear migration in fungi [24] , [25] . Indeed, dynein , LIS1 , NDEL1 and mammalian NUDC ( mNUDC ) are all nud genes [25] . Therefore, we also examined whether LC8 also stimulates disassembly of dynein–dynactin complex. Thus, two strong candidates, Arl3 and LC8, were selected and subjected to microtubule pull-down assays. Dynactin p150 Glued by itself is capable of direct binding to microtubules [10] . In addition, cytoplasmic dynein binds dynactin through a direct interaction between the DIC and p150 Glued (ref. 26 ). We examined whether the two candidates were able to release dynein from microtubule-bound dynactin under a high ATP condition, in which dynein was in a low-affinity state with microtubules [27] ( Supplementary Fig. 1c ). Without microtubules, the majority of dynein and dynactin was distributed in the supernatant fraction ( Fig. 1a lanes 1 and 2). When microtubules were added, a substantial fraction of dynein was distributed in the supernatant fraction without dynactin ( Fig. 1a lanes 3 and 4), whereas the presence of dynactin shifted dynein to the pellet fraction ( Fig. 1a lanes 5 and 6), suggesting that the increased population in the pellet was attributable to dynactin-bound dynein. Addition of the GTP-bound Arl3(Q71L) mutant significantly increased the proportion of dynein that was distributed in the supernatant fraction ( Fig. 1a lanes 7 and 8), while the addition of LC8 increased the proportion of dynein in the supernatant fraction ( Fig. 1a lanes 9 and 10). In contrast, a GDP-bound Arl3 mutant [28] Arl3(T31N) did not display any releasing properties ( Supplementary Fig. 1d ). Importantly, the combination of Arl3(Q71L) and LC8 enhanced the dissociation of dynein from dynactin ( Fig. 1a lanes 11 and 12). In contrast, Arl3(Q71L) and/or LC8 did not display any obvious effects on the interaction of dynactin and microtubules ( Fig. 1a lower panel). 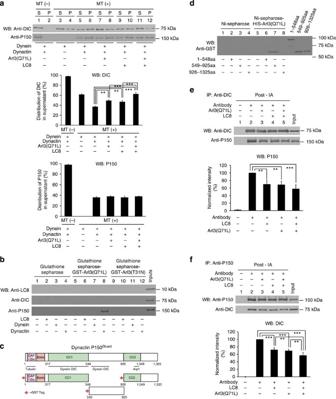Figure 1: Effect of Arl3(Q71L) and LC8 on dynein–dynactin interaction. (a) Microtubule pull-down assays using purified cytoplasmic dynein, dynactin and recombinant proteins: Arl3(Q71L) and LC8. After microtubule pull-down assay performed with or without microtubules, supernatants (S) and pellets (P) were analysed by WB for examination of the change in the ratio of dynein and dynactin. Upper WB: addition of Arl3(Q71L) or LC8 increased dynein amounts in the supernatant (lanes 5–10). Addition of both Arl3(Q71L) and LC8 simultaneously (lanes 11 and 12) resulted in the significant increase of dynein in the supernatant. However, addition of Arl3(Q71L) and/or LC8 did not affect dynactin binding to microtubules (lower panel). Lower graphs: the change of the ratios of dynein (left) or dynactin (right) in the supernatant were quantified (n=5). (b) GST pull-down assay; 0.4 μM Arl3(Q71L) or Arl3(T31N) prebound to glutathione sepharose were reacted with 0.5 μM dynein, dynactin and LC8, respectively (lanes 5–12). As shown in lanes 5–8, Arl3(Q71L) bound to dynactin, but not to dynein or LC8. Input lane indicates 10% of each protein used for GST pull-down assay. (c) Schematic diagram of P150Gluedsubunit of dynactin with previously mapped interaction sites. Three GST-tagged P150Gluedfragments were used ind. (d) HIS pull-down experiments. As shown here, P150Gluedfragment aa 549–925 was bound to Arl3(Q71L). Input lanes indicate 10% of each protein used. (e,f) Immunoprecipitation (IP) assays. Intrinsic Arl3- and LC8-depleted MEF cell lysates (Supplementary Fig. 1g,h) were immunoprecipitated with an anti-DIC (e) or -P150Gluedantibody (f). Precipitates were treated with Arl3(Q71L) or LC8 alone or in combination. Ine, co-precipitated dynactin was apparently reduced after addition of Arl3(Q71L) or LC8 alone, especially in together (lanes 2–5). Similarly, infthe amount of co-precipitated dynein was significantly reduced by addition of Arl3(Q71L) or LC8 alone or in combination (lanes 2–5). Input lane indicates 5% of cell extract used for immunoprecipitation assay. Lower quantitative graphs (n=4) indicate the reduction of co-precipitated proteins.P-values were calculated using analysis of variance, mean±s.e., **P<0.01, ***P<0.001. Figure 1: Effect of Arl3(Q71L) and LC8 on dynein–dynactin interaction. ( a ) Microtubule pull-down assays using purified cytoplasmic dynein, dynactin and recombinant proteins: Arl3(Q71L) and LC8. After microtubule pull-down assay performed with or without microtubules, supernatants (S) and pellets (P) were analysed by WB for examination of the change in the ratio of dynein and dynactin. Upper WB: addition of Arl3(Q71L) or LC8 increased dynein amounts in the supernatant (lanes 5–10). Addition of both Arl3(Q71L) and LC8 simultaneously (lanes 11 and 12) resulted in the significant increase of dynein in the supernatant. However, addition of Arl3(Q71L) and/or LC8 did not affect dynactin binding to microtubules (lower panel). Lower graphs: the change of the ratios of dynein (left) or dynactin (right) in the supernatant were quantified ( n =5). ( b ) GST pull-down assay; 0.4 μM Arl3(Q71L) or Arl3(T31N) prebound to glutathione sepharose were reacted with 0.5 μM dynein, dynactin and LC8, respectively (lanes 5–12). As shown in lanes 5–8, Arl3(Q71L) bound to dynactin, but not to dynein or LC8. Input lane indicates 10% of each protein used for GST pull-down assay. ( c ) Schematic diagram of P150 Glued subunit of dynactin with previously mapped interaction sites. Three GST-tagged P150 Glued fragments were used in d . ( d ) HIS pull-down experiments. As shown here, P150 Glued fragment aa 549–925 was bound to Arl3(Q71L). Input lanes indicate 10% of each protein used. ( e , f ) Immunoprecipitation (IP) assays. Intrinsic Arl3- and LC8-depleted MEF cell lysates ( Supplementary Fig. 1g,h ) were immunoprecipitated with an anti-DIC ( e ) or -P150 Glued antibody ( f ). Precipitates were treated with Arl3(Q71L) or LC8 alone or in combination. In e , co-precipitated dynactin was apparently reduced after addition of Arl3(Q71L) or LC8 alone, especially in together (lanes 2–5). Similarly, in f the amount of co-precipitated dynein was significantly reduced by addition of Arl3(Q71L) or LC8 alone or in combination (lanes 2–5). Input lane indicates 5% of cell extract used for immunoprecipitation assay. Lower quantitative graphs ( n =4) indicate the reduction of co-precipitated proteins. P -values were calculated using analysis of variance, mean±s.e., ** P <0.01, *** P <0.001. Full size image Previous work revealed that LC8 binds to DIC [29] , [30] , but the binding partner of Arl3 is unknown. To examine whether Arl3 binds either dynein, dynactin or LC8, we performed glutathione S -transferase (GST) pull-down assays using Arl3-conjugated beads. Dynactin was specifically precipitated with Arl3(Q71L)-conjugated beads ( Fig. 1b lanes 5 and 8), while Arl3(T31N) did not display obvious interactions with either dynein, dynactin or LC8 ( Fig. 1b lanes 9–12). We conclude that dynactin is a target molecule of Arl3. In contrast, we were not able to detect direct interaction between p150 Glued and LC8 ( Supplementary Fig. 1e ). To better understand the cargo unloading mechanism, we further examined the Arl3-binding domain on p150 Glued . We performed histidine (HIS) pull-down experiments using a series of bacterially expressed GST-tagged p150 Glued constructs ( Fig. 1c ). Interestingly, Arl3 specifically bound to the domain located between two CC domains ( Fig. 1d ). We next performed immunoprecipitation assays using cell lysates from cultured MEF cell after adding Arl3(Q71L) and LC8 recombinant proteins ( Fig. 1e,f and Supplementary Fig. 1f–h ). To precisely evaluate Arl3 and LC8 effects, we depleted endogenous Arl3 and LC8 by immunoabsorption ( Supplementary Fig. 1g,h ) and performed an immunoprecipitation assay. We precipitated dynein complexes by an anti-DIC antibody and found that p150 Glued co-precipitated with dynein ( Fig. 1e lane 2). Importantly, the amount of p150 Glued co-precipitation was significantly decreased in the presence of either Arl3(Q71L) or LC8 ( Fig. 1e : lanes 3 and 4). The combination of Arl3(Q71L) and LC8 further decreased p150 Glued co-precipitation ( Fig. 1e lane 5). We also precipitated dynein complexes with an anti-p150 Glued antibody and found that dynein co-precipitated with dynactin ( Fig. 1f lane 2). As in the previous experiment, the amount of DIC co-precipitation with anti-P150 Glued was significantly decreased in the presence of either Arl3(Q71L) or LC8 ( Fig. 1f lanes 3 and 4). Furthermore, the combination of Arl3(Q71L) and LC8 resulted in more significant reduction of DIC co-precipitation ( Fig. 1f lane 5). The use of endogenous Arl3- and LC8-depleted cell lysates ( Supplementary Fig. 1g,h ) exhibited consistent results of immunoprecipiation with the microtubule pull-down assay ( Fig. 1a ). Thus, we concluded that both Arl3(Q71L) and LC8 are key molecules for the negative regulation of dynein–dynactin interaction. Release of dynactin from dynein in vitro To obtain further evidence for Arl3(Q71L)- or LC8-mediated dissociation of dynactin from dynein, we performed in vitro single-molecule assays using purified dynein, dynactin, as well as recombinant proteins of Arl3(Q71L) and LC8. To visualize the release of dynactin, we used quantum dots (Qdots) as extremely photostable fluorescent probes [20] . Dynein was linked to 655 Qdot using an antibody (clone: 74.1) to DIC, which was covalently bound to the surface of 655 nm Qdot by an EDAC ( N -(3-dimethylaminopropyl)- N ′-ethylcarbodiimide hydrochloride) coupling reaction. Traces of dynein movement were found, reproducing our previously published results [20] ( Supplementary Movie 1 ), in which 30% (321 out of 1,076) of Qdot-conjugated dynein was mobile. In following experiments, we only analysed mobile dynein particles that have potential normal structure and function. We next traced the movement of a dynein–dynactin complex using a dual-colour Qdot approach. Dynactin was linked to 605 Qdot using an anti-dynactin p150 Glued antibody. Dynein and dynactin frequently co-migrated without any effect on the velocity and processivity [31] , suggesting that dynein and dynactin made a stable complex ( Supplementary Fig. 2a and Supplementary Movie 2 ), and 51% (102 out of 201) of mobile dynein co-migrated with dynactin. We also traced the movement of a dynein–LC8 complex using a dual-colour Qdot approach. LC8 was linked to 705 Qdot using an anti-GST antibody, which recognized the GST tag that was conjugated to the N terminus of LC8. Dynein and LC8 also frequently co-migrated without affecting the velocity and processivity ( Supplementary Fig. 2b and Supplementary Movie 3 ), and 65% (413 out of 632) of mobile dynein co-migrated with LC8. We finally examined binding of Arl3(Q71L) and dynactin using this dual-colour Qdot approach. Arl3(Q71L) was linked to 705 Qdot using an anti-HIS antibody, which recognized the HIS tag that was conjugated to the N terminus of Arl3(Q71L). We found frequent co-localization of Arl3(Q71L) and dynactin ( Supplementary Fig. 2c ). To probe the effect of Arl3(Q71L) or LC8 on the dynein–dynactin complex, we examined whether Arl3(Q71L) or LC8 was able to release dynactin from the dynein motor using a triple colour Qdot approach [20] . We initially made moving complexes of dynein and dynactin, and then added either Arl3(Q71L) or LC8. Arl3(Q71L) formed a transient triple complex and co-migrated, which was followed by the dissociation of a dynactin–Arl3(Q71L) complex, resulting in dynein moving alone ( Fig. 2a , Supplementary Fig. 2d and Supplementary Movie 4 ). On the other hand, LC8 behaved differently from Arl3. Initially, a transient triple complex was formed, which co-migrated and then released dynactin alone, followed by dynein-LC8 co-migration ( Fig. 2b , Supplementary Fig. 2e and Supplementary Movie 5 ). We next wanted to examine the effect of Arl3(Q71L) and LC8 on the dynein–dynactin interaction, but the use of quadruple colour Qdot system was technically challenging. Therefore, we examined the effect of Arl3(Q71L) and LC8 on the dynein–dynactin interaction using a dual-colour Qdot system. Dynein and dynactin formed stable complexes ( Fig. 2c leftmost panel). The addition of Arl3(T31N) did not exhibit obvious effects on the dynein–dynactin complex ( Fig. 2c second panel). In contrast, the addition of either Arl3(Q71L) or LC8 resulted in a significant decrease in the population of dynein–dynactin complexes ( Fig. 2c third and fourth panels). Furthermore, in the presence of Arl3(Q71L) and LC8, dynein-dynactin complexes were further decreased ( Fig. 2c rightmost panel). These findings imply that Arl3(Q71L) and LC8 target dynactin and dynein, respectively, and facilitate dissociation of dynactin from the dynein motor. 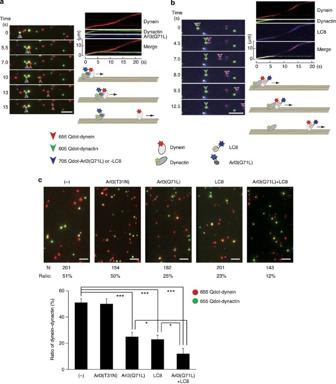Figure 2: Demonstration of dynactin release from a dynein–dynactin complex by anin vitrosingle-molecule assay. (a) Tracing Arl3(Q71L) interaction with dynein–dynactin complex by TIRF imaging. Arl3(Q71L) (705 Qdot conjugated, blue) appeared to provisionally bind to the dynein (655 Qdot conjugated, red)–dynactin (605 Qdot conjugated, green) complex and dissociated dynactin from dynein, arresting the dynactin-Arl3(Q71L) dimer on the microtubule as shown in the schematic diagrams (Supplementary Fig. 2dandSupplementary Movie 4). After dynactin dissociation, dynein continuously moved along the microtubule (Supplementary Movie 4). Individual kymographs represent dynein (red line), dynactin (green line), Arl3(Q71L) (blue line) and their merged image. (b) Unlike Arl3(Q71L), LC8 (705 Qdot conjugated, blue) appeared to temporarily bind to dynein–dynactin complex and detached dynactin from the dynein motor by forming a dynein-LC8 dimer as shown in the schematic diagrams (Supplementary Fig. 2eandSupplementary Movie 5). Thus, LC8 binds to dynein followed by co-migration with dynein motor (Supplementary Movie 5). The individual kymograph patterns of dynein, dynactin, LC8 (Blue line) and their merged image were shown in right side. Red, green and blue arrowheads indicate dynein, dynactin and Arl3(Q71L) or LC8, respectively. Scale bar, 5 μm (in montages); horizontal axis in the kymograph indicates moving time of Qdots, vertical axis in the kymograph indicates migration length of Qdots. (c) Effect of Arl3(Q71L) and LC8 on dynein–dynactin interaction using dual-colour Qdot approach. After addition of either Qdot unlabelled Arl3(T31N), Arl3(Q71L) or LC8 alone, or both Arl3(Q71L) and LC8 simultaneously, particles of moving dynein and dynein–dynactin complex were counted and the ratio of dynein–dynactin complexes was calculated as shown in the middle. The lower quantitative histogram represents the ratio of moving dynein–dynactin complex per moving dynein particles. Moving dynein–dynactin particles were decreased by addition of Arl3(Q71L) or LC8, especially when added together. In contrast, there was no detectable effect by addition of Arl3(T31N). Red, green and yellow colours indicate 655 Qdot-dynein, 605 Qdot-dynactin and dual-colour Qdot–dynein–dynactin complex, respectively. N, counted numbers of moving dynein particles from ten independent movies in each experiment; Ratio, ratio of moving dynein–dynactin complexes per moving dynein particles; scale bar, 5 μm. Figure 2: Demonstration of dynactin release from a dynein–dynactin complex by an in vitro single-molecule assay. ( a ) Tracing Arl3(Q71L) interaction with dynein–dynactin complex by TIRF imaging. Arl3(Q71L) (705 Qdot conjugated, blue) appeared to provisionally bind to the dynein (655 Qdot conjugated, red)–dynactin (605 Qdot conjugated, green) complex and dissociated dynactin from dynein, arresting the dynactin-Arl3(Q71L) dimer on the microtubule as shown in the schematic diagrams ( Supplementary Fig. 2d and Supplementary Movie 4 ). After dynactin dissociation, dynein continuously moved along the microtubule ( Supplementary Movie 4 ). Individual kymographs represent dynein (red line), dynactin (green line), Arl3(Q71L) (blue line) and their merged image. ( b ) Unlike Arl3(Q71L), LC8 (705 Qdot conjugated, blue) appeared to temporarily bind to dynein–dynactin complex and detached dynactin from the dynein motor by forming a dynein-LC8 dimer as shown in the schematic diagrams ( Supplementary Fig. 2e and Supplementary Movie 5 ). Thus, LC8 binds to dynein followed by co-migration with dynein motor ( Supplementary Movie 5 ). The individual kymograph patterns of dynein, dynactin, LC8 (Blue line) and their merged image were shown in right side. Red, green and blue arrowheads indicate dynein, dynactin and Arl3(Q71L) or LC8, respectively. Scale bar, 5 μm (in montages); horizontal axis in the kymograph indicates moving time of Qdots, vertical axis in the kymograph indicates migration length of Qdots. ( c ) Effect of Arl3(Q71L) and LC8 on dynein–dynactin interaction using dual-colour Qdot approach. After addition of either Qdot unlabelled Arl3(T31N), Arl3(Q71L) or LC8 alone, or both Arl3(Q71L) and LC8 simultaneously, particles of moving dynein and dynein–dynactin complex were counted and the ratio of dynein–dynactin complexes was calculated as shown in the middle. The lower quantitative histogram represents the ratio of moving dynein–dynactin complex per moving dynein particles. Moving dynein–dynactin particles were decreased by addition of Arl3(Q71L) or LC8, especially when added together. In contrast, there was no detectable effect by addition of Arl3(T31N). Red, green and yellow colours indicate 655 Qdot-dynein, 605 Qdot-dynactin and dual-colour Qdot–dynein–dynactin complex, respectively. N, counted numbers of moving dynein particles from ten independent movies in each experiment; Ratio, ratio of moving dynein–dynactin complexes per moving dynein particles; scale bar, 5 μm. Full size image Co-migration of dynactin/Arl3(Q71L) or dynein/LC8 in vivo To explore in vivo interaction of Arl3(Q71L) and LC8 with dynactin and dynein, respectively, we applied total internal reflection fluorescence (TIRF) microscopy to trace their movement in MEF cells. Indeed, both EGFP-p150 Glued and mCherry-Arl3 exhibited a punctate appearance in the perinuclear region ( Fig. 3a , Supplementary Fig. 3a and Supplementary Movie 6 ). Importantly, mCherry-Arl3(Q71L) displayed clear co-migration with EGFP-p150 Glued ( Fig. 3a , Supplementary Fig. 3a and Supplementary Movie 6 ). We focused on this motile population and analysed the mean square displacement (MSD) of single-particle traces as a function of the time lagΔ t (that is, the difference between two time points) [32] . 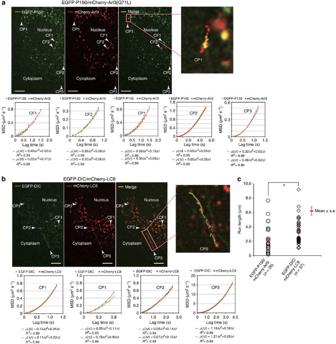Figure 3: Demonstration of co-migration of DIC and LC8, and P150Gluedand Arl3 at the centre of MEF cells by TIRF. (a) Representative traces in the MEF cells by TIRF microscopy expressing EGFP-P150Gluedand mCherry-Arl3 (upper panel,Supplementary Fig. 3a). White arrowheads indicate each starting point and direction for the centripetal (CP1–CP3) or centrifugal (CF1, CF2) migrations. MSDs were calculated from the motility of EGFP-P150Gluedand mCherry-Arl3 (lower panel,Supplementary Fig. 3a). Note: mCherry-Arl3 co-migrated with EGFP-P150Gluedin a centripetal and a centrifugal fashion. Enlarged image shown in right side is one of the traces (b) Representative traces in the MEF cells by TIRF microscopy expressing EGFP-DIC and mCherry-LC8 (upper panel,Supplementary Fig. 3b). White arrowheads indicate each starting point and direction for the centripetal (CP1–CP3) or centrifugal (CF1) migrations. MSDs were calculated from the motility of EGFP-DIC and mCherry-LC8 (lower panel,Supplementary Fig. 3b). Note: mCherry-LC8 co-migrated with EGFP-DIC in a centripetal and a centrifugal manner. Enlarged image shown in right side is one of the traces. Traces of EGFP-P150Glued, mCherry-Arl3, EGFP-DIC and mCherry-LC8 fit the second-order polynomial,ρ(Δt)=ν2Δt2+2DΔt+ζ (noise), indicating that they are following ballistic scaling behaviour rather than diffusive scaling behaviour. (c) Run length of EGFP-P150Glued/mCherry-Arl3 and EGFP-DIC/mCherry-LC8 were measured and summarized in a graph. Mean value of each combination was shown in red colour. CF, centrifugal migration; CP, centripetal migration;D, diffusion coefficient; TIRF; total internal reflection fluorescence;ν; mean velocity. Scale bar, 5 μm. The MSDs were plotted and fitted by two equations Figure 3: Demonstration of co-migration of DIC and LC8, and P150 Glued and Arl3 at the centre of MEF cells by TIRF. ( a ) Representative traces in the MEF cells by TIRF microscopy expressing EGFP-P150 Glued and mCherry-Arl3 (upper panel, Supplementary Fig. 3a ). White arrowheads indicate each starting point and direction for the centripetal (CP1–CP3) or centrifugal (CF1, CF2) migrations. MSDs were calculated from the motility of EGFP-P150 Glued and mCherry-Arl3 (lower panel, Supplementary Fig. 3a ). Note: mCherry-Arl3 co-migrated with EGFP-P150 Glued in a centripetal and a centrifugal fashion. Enlarged image shown in right side is one of the traces ( b ) Representative traces in the MEF cells by TIRF microscopy expressing EGFP-DIC and mCherry-LC8 (upper panel, Supplementary Fig. 3b ). White arrowheads indicate each starting point and direction for the centripetal (CP1–CP3) or centrifugal (CF1) migrations. MSDs were calculated from the motility of EGFP-DIC and mCherry-LC8 (lower panel, Supplementary Fig. 3b ). Note: mCherry-LC8 co-migrated with EGFP-DIC in a centripetal and a centrifugal manner. Enlarged image shown in right side is one of the traces. Traces of EGFP-P150 Glued , mCherry-Arl3, EGFP-DIC and mCherry-LC8 fit the second-order polynomial, ρ (Δ t )= ν 2 Δ t 2 +2 D Δ t +ζ (noise), indicating that they are following ballistic scaling behaviour rather than diffusive scaling behaviour. ( c ) Run length of EGFP-P150 Glued /mCherry-Arl3 and EGFP-DIC/mCherry-LC8 were measured and summarized in a graph. Mean value of each combination was shown in red colour. CF, centrifugal migration; CP, centripetal migration; D , diffusion coefficient; TIRF; total internal reflection fluorescence; ν ; mean velocity. Scale bar, 5 μm. Full size image and where D is the diffusion coefficient and ν is the mean velocity. If the particles of mCherry-Arl3(Q71L) or EGFP-p150 Glued move in a directed constant-velocity manner, that is, a ballistic scaling behaviour towards the transporting direction, the MSD would be fitted by equation (1), whereas if they move in purely random uncorrelated manner, the MSD would be fitted by equation (2). Fitting analysis revealed that the MSDs of mCherry-Arl3(Q71L) or EGFP-p150 Glued ( n =10) clearly fitted to Δ t 2 , suggesting that they behaved in a ballistic scaling manner (mean velocity±s.d. EGFP-p150 Glued : 0.62±0.45 μm s −1 , mCherry-Arl3(Q71L): 0.64±0.45 μm s −1 , Fig. 3a , Supplementary Fig. 3a and Supplementary Movie 6 ) [23] . We next applied TIRF microscopy to trace EGFP-DIC and mCherry-LC8. EGFP-DIC and mCherry-LC8 displayed co-migration in the perinuclear region ( Fig. 3b , Supplementary Fig. 3b and Supplementary Movie 7 ). The MSDs of EGFP-DIC and mCherry-LC8 ( n =11) also fitted to Δ t 2 , suggesting that they displayed ballistic scaling behaviour (mean velocity±s.d., EGFP-DIC: 0.68±0.38 μm s −1 , mCherry-LC8: 0.72±0.40 μm s −1 , Fig. 3b , Supplementary Fig. 3b and Supplementary Movie 7 ). Thus, we concluded that Arl3(Q71L) and LC8 bind dynactin and dynein in vivo , respectively. We examined run length of co-migration of each combination, which is summarized in Fig. 3c . Interestingly, DIC–LC8 complexes (mean run length±s.d. : 3.4 μm, n= 37) were prone to migrate longer distances than p150 Glued –Arl3 complexes (mean run length±s.d. : 2.2 μm, n= 26, Fig. 3c ). We interpret this to indicate that after binding of Arl3 to p150 Glued , the p150 Glued –Arl3 complex disassembled from a dynein motor, resulting in Brownian motion instead of ballistic motion, which leads to it passing out of the focus of a TIRF microscopy. Dynein and dynactin behaviours in Arl3- and/or LC8-KD cells The clear prediction from our model is that loss of Arl3 and LC8 function should result in the failure to unload cargoes from dynein motor at the minus end of microtubules. To address this prediction, we performed small interfering RNA (siRNA)-mediated Arl3 and LC8 knockdown experiments. In MEF cells, endogenous Arl3 and LC8 exhibited a gradient distribution carrying a peak at the perinuclear region ( Supplementary Fig. 4a ). In addition, this distribution overlapped with the distributions of p150 Glued and DIC, respectively, ( Supplementary Fig. 4b ). siRNAs against Arl3 or LC8 effectively depleted endogenous target proteins ( Fig. 4a–c ). After depletion of Arl3 or LC8, we found aberrant accumulation of dynein at the perinuclear region ( Fig. 4d upper paneland Fig. 4e ), which was confirmed by a quantitative analysis of fluorescence intensity ( Fig. 4g left). This aberrant distribution of dynein was rescued by enhanced green fluorescent protein (EGFP)-tagged human Arl3 (EGFP-hArl3) or human LC8 (EGFP-hLC8, Supplementary Fig. 4c–f ). Aberrant perinuclear distribution of dynactin was also observed after depletion of Arl3 or LC8 ( Fig. 4d lower panel and Fig. 4f,g right). Furthermore, dual depletion of Arl3 and LC8 exacerbated the perinuclear distribution of dynein and dynactin ( Fig. 4d rightmost panels and Fig. 4e–g ). We next determined the localization of membranous apparatuses after depletion of Arl3 and/or LC8. Early endosome antigen 1 (EEA1) and transferrin receptor (TfR) were used as markers of early and late endosomes, respectively [33] , [34] . Intracellular movement of mitochondria is also accomplished by microtubule-based motors [35] . Our results demonstrated that EEA1, TfR and mitochondria were abnormally accumulated in the perinuclear region by depletion of Arl3 or LC8 ( Fig. 5a,c ). Dual depletion of Arl3 and LC8 exhibited further profound effects on their localizations ( Fig. 5a rightmost panels and Fig. 5c ). This is consistent with our prediction that failure in unloading of cargoes inhibits the recycling of dynein and dynactin [4] , consequently resulting in the perinuclear accumulation of these membranous apparatuses. 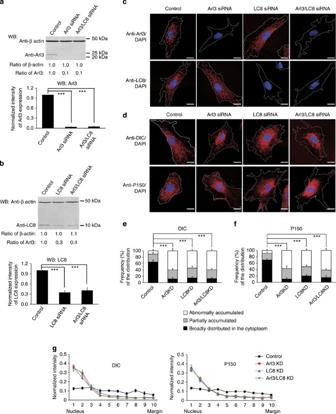Figure 4: Aberrant distribution of dynein or dynactin in Arl3- and/or LC8-depleted MEF cells. (a,b) SiRNA-mediated KD of Arl3 and/or LC8. Each siRNA-transfected MEF cell lysates were analysed by WB using antibodies against Arl3, LC8 and β-actin. Lower quantitative graphs show that siRNA treatment effectively decreased Arl3 or LC8 expression in both cases. β-Actin was used as loading control, samples prepared from three independent experiments. (c) Arl3 or LC8 alone or both siRNA-treated cells were probed with antibodies against Arl3 (upper panel) and LC8 (lower panel). Two kinds of siRNAs effectively inhibited expression of each target protein. (d) Localization of dynein and dynactin in each KD cells examined by using antibodies against DIC and P150Glued. Compared with control cells (leftmost panels), dynein (upper panel) and dynactin (lower panel) abnormally accumulated at the perinuclear region in all KD cells, especially in the dual KD cells (rightmost panels). (e,f) Quantitative data for aberrantly accumulated dynein (e) and dynactin (f). After siRNA treatment, the frequency of aberrantly accumulated dynein and dynactin at the perinuclear was analysed and compared with their control cells.P-values were from abnormally accumulated dynein or dynactin (n=100 cells, mean±s.e., ***P<0.001). (g) Quantified fluorescent intensity distribution of abnormally accumulated dynein (left) and dynactin (right) after depletion of Arl3 and/or LC8. As we previously reported (Yamadaetal., 2008, EMBO)49, fluorescent intensity along a linear line from the perinuclear area to the cell margin was measured and divided into ten compartments (horizontal axis) by the sum of the intensity in each region. Each fluorescence intensity measurement was corrected by subtraction of the background value. Intensity values in each graph were expressed mean±s.e., (n=10 cells). Cell nuclei were visualized with -4′, 6-diamidino-2-phenylindole (DAPI). Scale bar, 10 μm. IndicatedP-values were calculated using analysis of variance and data were expressed as mean±s.e., ***P<0.001. Figure 4: Aberrant distribution of dynein or dynactin in Arl3- and/or LC8-depleted MEF cells. ( a , b ) SiRNA-mediated KD of Arl3 and/or LC8. Each siRNA-transfected MEF cell lysates were analysed by WB using antibodies against Arl3, LC8 and β-actin. Lower quantitative graphs show that siRNA treatment effectively decreased Arl3 or LC8 expression in both cases. β-Actin was used as loading control, samples prepared from three independent experiments. ( c ) Arl3 or LC8 alone or both siRNA-treated cells were probed with antibodies against Arl3 (upper panel) and LC8 (lower panel). Two kinds of siRNAs effectively inhibited expression of each target protein. ( d ) Localization of dynein and dynactin in each KD cells examined by using antibodies against DIC and P150 Glued . Compared with control cells (leftmost panels), dynein (upper panel) and dynactin (lower panel) abnormally accumulated at the perinuclear region in all KD cells, especially in the dual KD cells (rightmost panels). ( e , f ) Quantitative data for aberrantly accumulated dynein ( e ) and dynactin ( f ). After siRNA treatment, the frequency of aberrantly accumulated dynein and dynactin at the perinuclear was analysed and compared with their control cells. P -values were from abnormally accumulated dynein or dynactin ( n =100 cells, mean±s.e., *** P <0.001). ( g ) Quantified fluorescent intensity distribution of abnormally accumulated dynein (left) and dynactin (right) after depletion of Arl3 and/or LC8. As we previously reported (Yamada et al. , 2008, EMBO) [49] , fluorescent intensity along a linear line from the perinuclear area to the cell margin was measured and divided into ten compartments (horizontal axis) by the sum of the intensity in each region. Each fluorescence intensity measurement was corrected by subtraction of the background value. Intensity values in each graph were expressed mean±s.e., ( n =10 cells). Cell nuclei were visualized with -4′, 6-diamidino-2-phenylindole (DAPI). Scale bar, 10 μm. Indicated P -values were calculated using analysis of variance and data were expressed as mean±s.e., *** P <0.001. 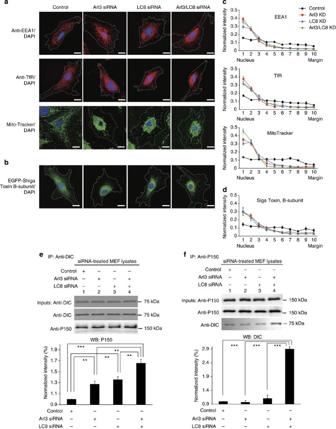Figure 5: Influences from impaired dynein–dynactin interaction caused by siRNA-mediated Arl3 and/or LC8 depletion in MEF cells. (a,b) Localization of membranous apparatuses in each KD cells examined by using antibodies against EEA1 and TfR, and Mito-Tracker and EGFP-Stx B-subunit. Compared with control cells (leftmost panels), early and late endosomes (a: upper and middle panels) abnormally accumulated at the perinuclear region in all KD cells, especially in the dual KD cells (rightmost panels). Similarly, mitochondria (a: lower panel) and EGFP-Stx B-subunit (b) also exhibited aberrant accumulation at the perinuclear region in all siRNA treated cells. Early and late endosomes were detected by antibodies against EEA1 and TfR, respectively. Cell nuclei were visualized with -4′, 6-diamidino-2-phenylindole (DAPI). Scale bar, 10 μm. (c,d) Quantified fluorescent intensity distribution of abnormally accumulated membranous apparatuses after depletion of Arl3 and/or LC8 (as described inFig. 4glegend). Intensity values in each graph were expressed mean±s.e., (n=10 cells). (e,f) Immunoprecipitation assay with an anti-DIC antibody (e) or an anti-P150Gluedantibody (f) using the cell extracts in which endogenous Arl3 and/or LC8 were depleted by siRNAs. Each input of cell extracts (5% of cell extract) and precipitates ineandfwere probed with anti-DIC or -P150Gluedantibody (upper two panels). Ine, compared with control (lane 1), depletion of endogenous Arl3 or LC8 led to significant increase of co-precipitation of dynactin (lanes 2 and 3), especially in dual depleted portion (lane 4). Inf, depletion of Arl3 or LC8 alone seems to have no apparent effect on dynein-dynactin interaction (lanes 1–3). In contrast, dual depletion of Arl3 and LC8 significantly increased co-precipitation of dynein (lane 4). Quantitative data and statistics are shown at the bottom. IndicatedP-values were calculated using analysis of variance and data were expressed as mean±s.e., **P<0.01, ***P<0.001. Full size image Figure 5: Influences from impaired dynein–dynactin interaction caused by siRNA-mediated Arl3 and/or LC8 depletion in MEF cells. ( a , b ) Localization of membranous apparatuses in each KD cells examined by using antibodies against EEA1 and TfR, and Mito-Tracker and EGFP-Stx B-subunit. Compared with control cells (leftmost panels), early and late endosomes ( a : upper and middle panels) abnormally accumulated at the perinuclear region in all KD cells, especially in the dual KD cells (rightmost panels). Similarly, mitochondria ( a : lower panel) and EGFP-Stx B-subunit ( b ) also exhibited aberrant accumulation at the perinuclear region in all siRNA treated cells. Early and late endosomes were detected by antibodies against EEA1 and TfR, respectively. Cell nuclei were visualized with -4′, 6-diamidino-2-phenylindole (DAPI). Scale bar, 10 μm. ( c , d ) Quantified fluorescent intensity distribution of abnormally accumulated membranous apparatuses after depletion of Arl3 and/or LC8 (as described in Fig. 4g legend). Intensity values in each graph were expressed mean±s.e., ( n =10 cells). ( e , f ) Immunoprecipitation assay with an anti-DIC antibody ( e ) or an anti-P150 Glued antibody ( f ) using the cell extracts in which endogenous Arl3 and/or LC8 were depleted by siRNAs. Each input of cell extracts (5% of cell extract) and precipitates in e and f were probed with anti-DIC or -P150 Glued antibody (upper two panels). In e , compared with control (lane 1), depletion of endogenous Arl3 or LC8 led to significant increase of co-precipitation of dynactin (lanes 2 and 3), especially in dual depleted portion (lane 4). In f , depletion of Arl3 or LC8 alone seems to have no apparent effect on dynein-dynactin interaction (lanes 1–3). In contrast, dual depletion of Arl3 and LC8 significantly increased co-precipitation of dynein (lane 4). Quantitative data and statistics are shown at the bottom. Indicated P -values were calculated using analysis of variance and data were expressed as mean±s.e., ** P <0.01, *** P <0.001. Full size image The AB 5 -subunit bacterial toxins, typified by cholera and Shiga toxin (Stx), enter host cells by moving retrogradely in the secretory pathway from the plasma membrane to the endoplasmic reticulum (ER), where it is then translocated to the cytosol to exert its toxic effect by inactivating ribosomes [36] . As the short B fragment of Shiga toxin is sufficient for transport to the ER, a GFP-tagged B-subunit can be used to trace the secretory pathway after endocytosis. In this secretory pathway, both anterograde and retrograde transports are required. Therefore, we examined whether depletion of Arl3 or LC8 affects endocytosis followed by dynein-mediated retrograde transport using EGFP-tagged Stx B-subunit (EGFP–B-subunit). Fluorescence microscopic analysis revealed that substantial amounts of the EGFP–B-subunit were incorporated into the cell, indicating that endocytosis of the EGFP–B-subunit was fairly intact regardless of depletion of Arl3 or LC8 ( Fig. 5b leftmost and Fig. 5d ). Importantly, the EGFP–B-subunit was prone to localize at the Golgi region by depletion of Arl3 or LC8 ( Fig. 5b middle two panelsand Fig. 5d ), especially in cells where both Arl3 and LC8 were depleted ( Fig. 5b rightmost and Fig. 5d ), suggesting that the transition from retrograde transport to anterograde transport was specifically impaired by depletion of Arl3 and/or LC8. We interpreted these findings to indicate that depletion of Arl3 and/or LC8 impaired release of the EGFP–B-subunit from dynein and affected its transfer to kinesin, resulting in the defective redistribution from the Golgi apparatus to ER. From these results, another interesting hypothesis emerged that reduction of Arl3 and/or LC8 should lead to increase dynein–dynactin association. To examine this prediction, endogenous Arl3- and/or LC8-depleted cell extracts by siRNAs were subjected to immunoprecipitation. Compared with control, the amount of p150 Glued co-precipitated with dynein was significantly increased by depletion of endogenous Arl3 or LC8 ( Fig. 5e lanes 1–3). Importantly, dual depletion further augmented the amount of co-precipitated dynactin ( Fig. 5e lane 4). On the other hand, in the case of immunoprecipitation using an anti-P150 Glued antibody, depletion of Arl3 alone seems to have no apparent effects on the dynein–dynactin interaction, whereas depletion of LC8 alone weakly increased the dynein–dynactin interaction ( Fig. 5f lanes 1–3). Although the reason of this difference is not clear, importantly, dynein co-precipitation was significantly increased by the dual depletion of Arl3 and LC8 ( Fig. 5f lane 4). As we expected, depletion of Arl3 and/or LC8 resulted in defective disassembly of dynactin from dynein, thereby resulting in increased dynein–dynactin association in MEF cells. These results would provide a new evidence to support our microtubule pull-down and immunoprecipitation assays ( Fig. 1a,e,f ), as well as the abnormally accumulated molecules and membranous apparatuses at the perinuclear region caused by siRNA treatment ( Figs 4d–g and 5a–d ). Taken together, our findings indicate that Arl3 and LC8 induce dissociation of dynactin from dynein, and consequently regulate unloading of cargoes from dynein motors. The regulation of assembly and disassembly of dynein–dynactin complex is an essential cellular process mediating the traffic of many cargoes within the cell. In this paper we have uncovered the regulatory mechanism of dynein–dynactin dissociation, as well as the cargo unloading. Our findings revealed that Arl3 and LC8 bind dynactin and dynein, respectively, and facilitate dissociation of dynactin from dynein. Why is such a dual regulation mechanism required? For stable transport, dynein and dynactin must achieve a high-affinity interaction, whereas for efficient unloading, a dynein–dynactin interaction is required to be reversible. To solve this opposing problem, Arl3 and LC8 may work during unloading, a notion supported by the similar subceullar localization of Arl3 and LC8 ( Supplementary Fig. 4a ). Although independent disassembly by Arl3 and LC8 is also possible, dual regulation ensure a more secure dissociation. Indeed, dual depletion of Arl3 and LC8 exacerbated the aberrant distribution of dynein and dynactin ( Fig. 4d–g ), as well as the membranous apparatuses ( Fig. 5a–d ). We also determined that Arl3 specifically binds to the domain between the CC1 and CC2 of p150 Glued ( Fig. 1c,d ). Functional importance of this domain to binding with dynein DIC is controversial [11] , [12] , [13] . The mechanisms by which Arl3 binding to p150 Glued facilitates the disassembly of dynein–dynactin complex is unknown. Presumably, Arl3 binding to the inter-CC domain of P150 Glued may simply compete for dynein binding and/or may induce allosteric modification. Further study to uncover a mechanism that links their action in vivo will unwind exquisite regulation of the unloading from dynein motor. Recently, it was reported that phosphotidylinositol-4-phosphate negatively regulates the protein–protein interaction between the p150 Glued and the retromer component sorting nexin 6 (SNX6) [37] . In this study, siRNA-mediated depletion of Arl3 and LC8 exhibited not only the aberrant distributions of dynein and dynactin ( Fig. 4d–g ), but also in the membranous apparatuses ( Fig. 5a–d ), which are all known to be transported by the microtubule-based dynein motor. These abnormal accumulations of endosomes by depletion of Arl3 and/or LC8 were also tightly coupled to the aberrant distribution of dynein and dynactin. Remarkably, depletion of endogenous Arl3 and/or LC8 increased the association of dynein–dynactin in MEF cells ( Fig. 5e,f ). These results suggest that disconnection of dynein and dynactin may be the first step for cargo unloading. We also uncovered the role of LC8 in cargo unloading. LC8 was originally identified as the smallest subunit of axonemal dynein in Chlamydomonas [38] . Interestingly, the gene required for nuclear migration, nudG , encodes a homologue of LC8 (ref. 23 ). In the filamentous fungus Aspergillus nidulans , nud mutants have been isolated, including nudA , nudF , nudE , nudG and nudC [24] , [25] . nudA , nudF and nudE encode dynein HC, LIS1 and NDEL/NDE1, respectively. Mammalian NUDC is required for kinesin-1-mediated anterograde transport of dynein [39] . Presumably, mutation of LC8 will lead to impairment not only of the unloading of cargoes but also dynein recycling. The phenotypes that were observed in siRNA-mediated LC8 depletion support this notion. Improper distribution of cytoplasmic dynein accompanied by nudG mutation in Aspergillus nidulans may provide the explanation of the nuclear migration defect. Intraflagellar transport (IFT) is a term used to describe the bidirectional transport of non-membrane protein particles in the cilia. LC8 is integral components of the dynein that powers retrograde IFT [40] , [41] . Interestingly, Arl13 and Arl3 operate to maintain the stability of IFT particles during middle segment transport in Caenorhabditis elegans [42] and Arl3 specifically releases myristoylated ciliary cargo [43] . Furthermore, Arl3-null mice displayed typical ciliopathy phenotypes [44] . Thus, LC8 and Arl3 display intimate relationship in IFT and ciliogenesis. Our new findings against Arl3 and LC8 function on the dynein–dynactin dissociation may shed light on the common pathway for the regulation of transport in the cilia and cytoplasm. Vectors used for expression and recombinant proteins Complementary DNAs carrying the full-length open reading frames of each of the proteins were conjugated to pEGFP (Clonetech Laboratories, CA, USA) or monomeric Cherry (mCherry) vectors (Clonetech Laboratories). Recombinant proteins for LC8 and Arl3 (wild-type, Q71L and T31N) were generated using a bacterial expression system (Invitrogen) and pGEX-4T expression vector (GE Healthcare Lifesciences, UK). Protein purification was performed using Glutathione Sepharose 4B (GE Healthcare Lifesciences) according to the manufacturer’s recommendation. To remove GST tag, we treated recombinant proteins with thrombin (GE Healthcare Lifesciences), followed by absorption of thrombin by Benzamidine Sepharose 6B (GE Healthcare Lifesciences). Purification of proteins Porcine brain cytoplasmic dynein, dynactin and tubulin were purified as described [45] , [46] , [47] . The anion exchange column (HiTrap Q HP; GE Healthcare, Uppsala, Sweden) was used for separation of dynein and dynactin. All of three purified protein samples were flash frozen and cryopreserved in liquid nitrogen until they were used. Microtubule pull-down assay Tubulin (7.6 mg ml −1 ) was polymerized in BRB80 buffer (80 mM pipes-NaOH, pH6.8, 2 mM MgSO 4 , 1 mM EGTA) containing 10 mM GTP, and 100 μM Taxol was added to maintain microtubule polymerization. Dynein (0.5 μM)–dynactin (0.5 μM) mixture was mixed with Arl3(Q71L) (0.5 μM) or LC8 (0.5 μM) alone or in combination in BRB80 buffer containing 10 mM ATP with microtubules. Some of the samples were incubated in the absence or presence of microtubules without any of the recombinant proteins. After incubation for 5 min at room temperature, microtubules were centrifuged at 200,000 g for 10 min at room temperature using a 120.2 rotor in an Optima TLX ultracentrifuge (Beckman Coulter, CA, USA). The supernatants and pellets were separated and analysed by western blotting (WB) using anti-DIC (1,000 × dilution in this study) or -P150 Glued (1,000 × dilution in this study) antibody. Blotted membranes were quantified by LAS3000 (FUJI FILM, Tokyo, Japan). Immunoabsorption and immunoprecipitation Immunoprecipitation experiments were performed as described with a slight modification [48] . MEF cell pellets were resuspended in a homogenization buffer (20 mM Tris, pH 8.0, 0.1 M KCl, 1 mM phenylmethylsulphonyl fluoride, 5 μg ml −1 each of aprotinin, leupeptin and pepstatin A, 5 mM ATP, 1% Triton X-100) and vortexed before centrifugation. To remove endogenous Arl3 and LC8, cell lysates were collected and incubated with anti-Arl3 (Proteintech Group Inc., IL, USA) and -LC8 (Sigma-Aldrich) antibodies prebound to protein A-Sepharose (GE Healthcare Lifescience) for 2 h at 4 °C. Supernatant was further subjected to immunoprecipitation analysis as follows. Immunoabsorbed MEF lysates were continuously incubated with antibodies (anti-DIC (EMD Millipore, Darmstadt, Germany) or -P150 Glued (BD Biosciences, SJ, California)) prebound to protein G-Sepharose beads (GE Healthcare Lifescience) for 2 h at 4 °C. After incubation, cell lysates were removed completely, followed by addition of recombinant protein Arl3(Q71L) (0.5 μM) or LC8 (0.5 μM), or both of them. Finally, the beads were washed and the proteins were eluted in SDS–PAGE sample buffer and analysed by WB. EGFP-DIC-overexpressed MEF lysate was also subjected to immunoprecipitation to confirm the suitability of 74.1, the anti-DIC antibody in this approach. MEF lysates containing EGFP-DIC were treated with anti-EGFP antibody (JL-8, BD Biosciences) prebound to protein G-Sepharose before addition of target recombinants. Here, freshly prepared 2% BSA/1% casein was used as blocking buffer of sepharose. Original images of western blottings shown in Figs 1 and 5 are available in Supplementary Fig. 5 . In vitro single-molecule assay Single-molecule assays using a custom-built TIRF microscope were performed according to our previous work with slight modifications [20] . For labelling dynein and dynactin, 655 Qdot and 605 Qdot (emitting at 655 and 605 nm, respectively; Life Technologies, CA, USA) were cross-linked to anti-DIC antibody and anti-P150 Glued antibody respectively, via EDAC (Sigma-Aldrich), and then mixed with dynein (0.8 μM) or dynactin (0.8 μM). GST-tagged LC8 or HIS-tagged Arl3(Q71L) was labelled with 705 Qdot (emitting at 705 nm; Life Technologies) by using anti-GST antibody (Medical and Biological Laboratories, Nagoya, Japan) or anti-HIS antibody (Clontech, Mountain View, California). In the case of dual-colour Qdots-labelled dynein–dynactin complex, dynein and dynactin were premixed on ice for more than 30 min before addition of Qdots. We used a molar ratio between Qdot and target protein for all experiments of 1:1. Tubulin (7.6 mg ml −1 ) was polymerized in BRB80 buffer (80 mM pipes-NaOH, pH 6.8, 2 mM MgSO 4 , 1 mM EGTA) containing 10 mM GTP, and 50 μM Taxol was added to maintain microtubule polymerization. The observation chamber was coated with anti-α tubulin antibody (TU-02; Santa Cruz Biotechnology) and washed with blocking buffer (10 mg ml −1 casein). Then, polymerized microtubules in final dilution buffer (25 mM CH 3 COOK, 4 mM MgSO 4 , 1 mM EGTA, 10 mM Pipes-KOH, pH 7.0, 50 μM Taxol, oxygen scavenger (25 mM glucose, 216 μg ml −1 glucose oxidase, 36 μg ml −1 catalase and 10 mM dithiothreitol)) were loaded and fixed to the chamber. After removing unbound microtubules with blocking buffer, premixed Qdot-labelled dynein–dynactin complex with Arl3(Q71L) or LC8 were added to the chamber and incubated at 37 °C with a lens heater for 3 min. Excess Qdot-labelled target proteins were rinsed briefly with blocking buffer followed by flowing final dilution buffer supplemented with 10 mM ATP and immediately viewed by a 488-nm laser at 45 mW (Sapphire; Coherent, CA, USA). The split images were passed through each emission filter (Brightline; Semrock Inc., IL, USA) and captured simultaneously by an electron multiplying charge-coupled device camera (iXon; Andor Technology, Belfast, Northern Ireland). Time-lapse images were acquired at 100 ms intervals and further processed using ImageJ software (National Institutes of Health, MD, USA). Dual-colour Qdot-labelled dynein–dynactin complexes were also treated with Qdot-unlabelled Arl3(Q71L) (200 nM) and LC8 (200 nM). Unlabelled Arl3 or LC8 alone or both of them was mixed with dual-colour Qdot-labelled dynein–dynactin complex for 10 min on ice just before loading to an observation chamber. After capturing images, the frequency of dynein–dynactin complexes was calculated. In vivo single-molecule fluorescence imaging Both EGFP-DIC and mCherry-LC8 or both EGFP-P150 Glued and mCherry-Arl3 were co-expressed in MEFs using the Neon transfection system and excited simultaneously by 488 and 561 nm continuous wave mode lasers, respectively (Excelsior 488, 50 mW and Excelsior 561, 50 mW, Spectra-Physics, Inc., Tokyo, Japan). Fluorescence images were obtained using an inverted microscope (ECLIPSE T i , Nikon Instech Co., Tokyo, Japan) through an oil-immersion objective lens (Apo TIRF 100 × , numerical aperture 1.49, Nikon Instech Co., Tokyo, Japan). By using dual view optics (W-View A8509, Hamamatsu Photonics, Hamamatsu, Japan), each emission was split into two parts at 550 nm by a dichroic mirror (DM550LP and DM550SP, Hamamatsu Photonics). The split images were passed through an emission filter (FF01-525/45-25 for EGFP and FF01-609/54-25 for mCherry, Semrock Inc.) and captured simultaneously by a scientific complementary metal-oxide semiconductor camera (ORCA-Flash 4.0, Hamamatsu Photonics). All experiments were performed at 37 °C with a lens heater (Tokai-Hit, Shizuoka, Japan). For the single-particle tracking of EGFP or mCherry fusion proteins, the centres of MEFs were continuously observed. Time-lapse images were acquired at 100 ms intervals and further processed using ImageJ software (National Institutes of Health) with self-work particle-tracking plugins developed by Y.A. To further analyse the movement of fluorescent-labelled molecule, the MSD ( ρ (Δ t )) against time, which is a convenient for quantitative measure of stochastic movement, was calculated by R software. The MSD was plotted and fitted by two equations, ρ 2(Δ t )=2 D Δ t + ν 2 Δ t 2 +ζ (noise) and ρ 1(Δ t )=4 D Δ t +ζ (noise), where D is the diffusion coefficient, ν is the mean velocity and ζ is noise term. siRNAs and cell culture siRNAs targeted to the sequence of mouse Arl3: 5′-GCAUGAACUGGGUCUGCAATT-3′, mouse LC8: 5′-CCAAAUUCCAAAUACCAGATT-3′ and a firefly ( Photinus pyralis ) luciferase (pGL2) 5′-CGUACGCGGAAUACUUCGATT-3′ as a negative control were synthesized by Sigma-Aldrich (MO, USA). Each double-stranded 21-nucleotide RNA at a final concentration of 200–400 nM was transfected into the MEF cells using the Neon transfection system (Life Technologies). MEF cells were plated onto poly- L -lysine coated with or without glass based six-well plate (IWAKI Glass Inc., Tokyo, Japan) and cultured in D-MEM (Wako Chemicals, Osaka, Japan) with 10% heat-inactivated fetal bovine serum (Nichirei Biosciences, Tokyo, Japan) for 48 h before analysis. Arl3 and LC8 siRNA-treated MEF cells were also transfected with EGFP-hArl3 and EGFP-hLC8, respectively, as knockdown rescue controls. After 48 h of culturing, cells were analysed by WB or immunocytochemistry. Immunocytochemistry All MEFs used in this study were fixed with 4% ultra-pure electron microscopy-grade paraformaldehyde for 15 min at room temperature and permeabilized with 0.2% Triton X-100 for 10 min at room temperature. Cells were then blocked with 5% BSA and Block Ace Powder (DS Pharma Biomedical Co., Ltd, Osaka, Japan) in PBS and incubated with anti-Arl3 antibody (100 × dilution, Proteintech Group Inc.), anti-DYNLL1/LC8 antibody (100 × dilution, Sigma-Aldrich), anti-Dynein antibody, 74 kDa ICs (anti-DIC, EMD Millipore), anti-P150 Glued antibody (BD Biosciences), nti-EEA1 (100 × dilution, Abcam, Cambridge, UK) or anti-TfR receptor (100 × dilution, Life Technologies) followed by incubation with Alexa546-conjugated anti-mouse IgG or Alexa546-conjugated anti-rabbit IgG (2,000 × dilution, Life Technologies). Each incubation was performed for 1 h at room temperature. Anti-Arl3 antibody used in this study specifically recognized Arl3, without cross-reaction with Arl2. Slides were mounted in FluoSave Reagent (EMD Millipore) containing 100 nM 4′,6-diamidino-2-phenylindole (0.2 μM). The images were observed and captured with a laser scanning confocal microscope (LSM510META, Carl Zeiss, Oberkochen, Germany). EGFP-tagged Stx B-subunit trafficking in MEF Cell Recombinant protein of GST-fused EGFP-Stx B-subunit (EGFP–B-subunit) was expressed in bacteria and purified using Glutathione Sepharose 4B (GE Healthcare Lifesciences) according to the manufacturer’s recommendation. To remove GST tag, we treated recombinant proteins with thrombin (GE Healthcare Lifesciences), followed by absorption of thrombin by Benzamidine Sepharose 6B (GE Healthcare Lifesciences). MEF cells were incubated on ice with 2.5 μg ml −1 of EGFP–B-subunit in D-MEM without 10% FBS for 2 min. The cells were washed three times with fresh medium and incubated at 37 °C for 30 min with D-MEM (Wako Chemicals) with 10% heat-inactivated fetal bovine serum (Nichirei Biosciences, Tokyo, Japan). The distribution of EGFP–B-subunit was examined by confocal microscopy. Stx B-subunit plasmid was kindly provided by Dr Imai Yasuyuki (University of Shizuoka). How to cite this article: Jin, M. et al. Arl3 and LC8 regulate dissociation of dynactin from dynein. Nat. Commun. 5:5295 doi: 10.1038/ncomms6295 (2014).